Fossilized iron bacteria reveal a pathway to the biological origin of banded iron formation Debates on the formation of banded iron formations in ancient ferruginous oceans are dominated by a dichotomy between abiotic and biotic iron cycling. This is fuelled by difficulties in unravelling the exact processes involved in their formation. Here we provide fossil environmental evidence for anoxygenic photoferrotrophic deposition of analogue banded iron rocks in shallow marine waters associated with an Early Quaternary hydrothermal vent field on Milos Island, Greece. Trace metal, major and rare earth elemental compositions suggest that the deposited rocks closely resemble banded iron formations of Precambrian origin. Well-preserved microbial fossils in combination with chemical data imply that band formation was linked to periodic massive encrustation of anoxygenic phototrophic biofilms by iron oxyhydroxide alternating with abiotic silica precipitation. The data implicate cyclic anoxygenic photoferrotrophy and their fossilization mechanisms in the construction of microskeletal fabrics that result in the formation of characteristic banded iron formation bands of varying silica and iron oxide ratios. It is generally believed that banded iron formations (BIFs), the bulk of which was formed in the late Archaean/Palaeoproterozoic marine basins, occurred in stratified water columns deep in the ocean and on continental shelf margins [1] , [2] , [3] , [4] . Soluble ferrous iron, supplied from mid-ocean ridges and hydrothermal vents, was oxidized by various processes to ferric iron and deposited in association with varying silica ratios as BIFs [1] , [2] , [3] , [4] . But the mechanism that drove and sustained the massive and sporadic deposition of BIFs throughout much of the Precambrian remains a mystery, despite decades of research. The low Archaean oxygen levels (~10 −5 of present-day concentrations or even less [5] ) are generally considered insufficient to have supported broad-scale BIF generation [1] , [6] . Instead, biotic, anoxygenic photoferrotrophic precipitation according to the equation 4Fe 2+ +CO 2 +11H 2 O+light→[CH 2 O]+4Fe(OH) 3 +8H + has been proposed [6] , [7] , [8] , [9] , [10] , [11] , [12] , [13] , [14] . With the exemption of proxies such as iron isotopes [12] , [13] , there exists no direct environmental evidence—neither in ancient nor in modern ecosystems—demonstrating how photoferrotrophs could have accounted for vast-scale biological BIF deposition, including the formation of their spectacular banded consistency. Cape Vani, located on the NW of Milos Island, in the Hellenic (Aegean) Volcanic Arc, hosts an Early Quaternary shallow ferruginous marine microbial deposit that was supported by chemical energy released from focused and diffused hydrothermal vents [15] , [16] . Biogeochemical evidence indicates that this deposit occurred in a restricted shallow marine basin at the foot of an andesite continental shelf, where calm waters resulted in water column stratification and the development of local anoxia [15] . We provide new biogeochemical data supporting this fact and independently illustrate that these conditions resemble those that supported the deposition of some Precambrian BIFs, with the iron sourced from seafloor hydrothermal vents and hotspots. Geology and geochemistry The Cape Vani rocks ( Fig. 1 ; see Supplementary Fig. S1 for a description of the geology of the field site) display remarkable BIF-like patterns ( Fig. 2 ), including alternating micrometric to millimetric iron oxide and silica bands ( Supplementary Fig. S2 ). Similar to Precambrian BIFs, silica/iron ratios in these rocks are inversely related ( Fig. 3a ), while a low range of TiO 2 , Al 2 O 3 and K 2 O concentrations suggest little terrigenous sedimentary input [17] , [18] , [19] . Heavy rare earth element (REE) enrichment occurs in both the ferruginous and siliceous components of the rock relative to light REE ( Fig. 3b ) and is comparable to reported Precambrian BIF profiles [17] , [18] , [19] . Together with a pronounced positive Eu anomaly, these observations hint at a hydrothermal origin of the deposits as opposed to seawater-derived sediments that are often light REE-enriched relative to heavy rare earth elements [18] . Calculated Eu/Eu* and Ce/Ce* anomalies (North American Shale Composite (NASC) normalized) of ~0.23 and ~2.56, respectively, lie within the reported Precambrian BIF range, while Ce depletion in relation to the other REEs supports anoxic depositional conditions [17] , [18] , [19] . Sedimentary Ce levels are generally expected to increase under oxidizing conditions because, unlike most REEs, Ce 3+ is oxidized to Ce 4+ and coprecipitated in association with iron oxyhydro(oxides) [17] , [18] , [19] . Furthermore, the occurrence and preservation of MnO ( Fig. 3c ) in concentrations comparable to Mesoarchean Witwatersrand Supergroup BIFs [19] supports a reduced sedimentary environment. 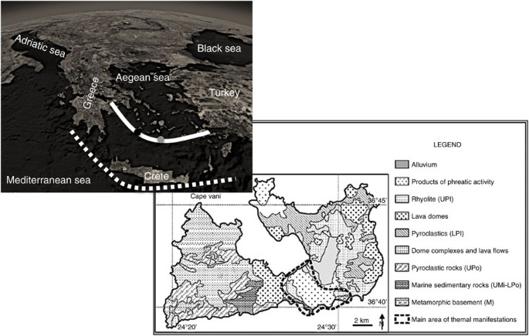Figure 1: Location and geologic features of Cape Vani. Inset, satellite map showing the location of Milos Island (black circle on unbroken white line). Grey circle on unbroken white line indicates Santorini. Broken white line shows the Hellenic Trench, where the African plate is subducted under the Euroasian plate to give rise to the Hellenic (Aegean) Volcanic Arc (unbroken white line). UPI—upper Pleistocene; LPI—lower Pleistocene; UPo—upper Pliocene; LPo—lower Pliocene; UMi—upper Miocene; M—Mesozoic (16). Figure 1: Location and geologic features of Cape Vani. Inset, satellite map showing the location of Milos Island (black circle on unbroken white line). Grey circle on unbroken white line indicates Santorini. Broken white line shows the Hellenic Trench, where the African plate is subducted under the Euroasian plate to give rise to the Hellenic (Aegean) Volcanic Arc (unbroken white line). UPI—upper Pleistocene; LPI—lower Pleistocene; UPo—upper Pliocene; LPo—lower Pliocene; UMi—upper Miocene; M—Mesozoic (16). 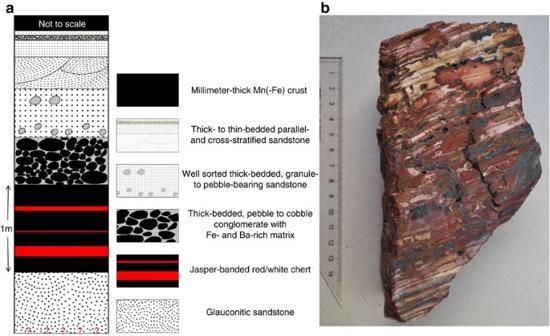Figure 2: Stratigraphy of the Cape Vani deposit. (a) The lithofacies association, constituting the fossiliferous Cape Vani-banded Fe-rich sedimentary chert, NW Milos Island. (b) Sawed rock sample of the investigated chert. Details are found inSupplementary Fig. S1. Full size image Figure 2: Stratigraphy of the Cape Vani deposit. ( a ) The lithofacies association, constituting the fossiliferous Cape Vani-banded Fe-rich sedimentary chert, NW Milos Island. ( b ) Sawed rock sample of the investigated chert. Details are found in Supplementary Fig. S1 . 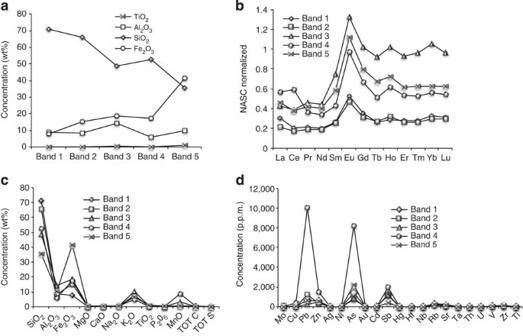Figure 3: Whole rock chemistry. (a) Behaviour of silica, haematite, Al2O3and TiO2. (b) NASC normalized REE fractionation profiles. Minimum detection limit (MDL) varied from 0.01 to 0.1 p.p.m. (c) Behaviour of major elements. MDL ranged from 0.002 for Cr2O3to 0.04 wt% for Fe2O3. Cr2O3was consistently below the detection limit. (d) Trace elemental composition. MDL varied from 0.1 to 1 p.p.m., with the exception of Ni that had an MDL of 20 p.p.m. and was below the MDL. Bi, Sn and Se were below MDL (0.1, 1, 0.5, respectively). Unusually high As and Pb concentrations (>8,000 and 10,000 p.p.m., respectively) were identified in the jaspers in banded 4, respectively. Full size image Figure 3: Whole rock chemistry. ( a ) Behaviour of silica, haematite, Al 2 O 3 and TiO 2 . ( b ) NASC normalized REE fractionation profiles. Minimum detection limit (MDL) varied from 0.01 to 0.1 p.p.m. ( c ) Behaviour of major elements. MDL ranged from 0.002 for Cr 2 O 3 to 0.04 wt% for Fe 2 O 3 . Cr 2 O 3 was consistently below the detection limit. ( d ) Trace elemental composition. MDL varied from 0.1 to 1 p.p.m., with the exception of Ni that had an MDL of 20 p.p.m. and was below the MDL. Bi, Sn and Se were below MDL (0.1, 1, 0.5, respectively). Unusually high As and Pb concentrations (>8,000 and 10,000 p.p.m., respectively) were identified in the jaspers in banded 4, respectively. Full size image Cr in oceanic sediments has been mostly associated with a terrigenous origin, resulting from the dissolution of ultramafic rocks and soils [20] , [21] . In oxygenated conditions, the released Cr 3+ is oxidized by Mn(III) and (IV) to stable Cr 6+ , which under reducing conditions is transformed by microbial activity and Fe 2+ to Cr 3+ and preserved in association with iron oxyhydro(oxides) [20] , [21] . Instead, we found that Cr 3+ was consistently below the detection limit, a situation similar to the low Cr 3+ concentrations reported for much of Archaean Agloma-type BIFs deposited close to deep submarine volcanic arcs and spreading ridges [21] . After ~2.5 Ga, superior-type BIF facies (near-shore continental shelf deposits) were reported to have experienced a sudden spike in Cr concentrations, which was linked to the clastic detrital input resulting from oxygen-driven weathering of crustal rocks [20] , [21] . Our Cr data thus support the idea of low oxygen tension in the water column, where the Cape Vani marine deposits were formed, with low levels of continental crust detrital delivery into the basin. The haematite signal varied in the Cape Vani deposits as a function of silica concentrations whereas trace elemental compositions followed the same general trends, regardless of the silica to iron ratio ( Fig. 3d ), indicating that the rocks were deposited under persistent/consistent biogeochemical conditions for extended periods. The high silica load particularly suggests an ocean saturated with hydrothermally derived amorphous silica, similar to the inferences made for Precambrian oceans from a chemical analysis of BIFs [1] , [17] , [18] . No organic carbon signal was obtained by Raman spectroscopy—a BIF feature often attributed to remineralization of organic matter to dissolved inorganic carbon through respiration [22] . The largely low levels of whole-rock total carbon supports this hypothesis, whereas the close to zero total sulphur concentrations suggest a non-sulphidic depositional environment ( Fig. 3c ). Therefore, the Cape Vani deposit could be classified as a cherty, low-carbon, haematite-rich BIF analogue, formed under reducing conditions. The recorded low oxygen concentrations would have promoted anaerobic chemoautotrophic iron oxidation [19] . Fossil iron bacteria From the haematite-rich jasper bands ( Fig. 2 and Supplementary Fig. S2 ) we report remarkably well-preserved microbial fossils ( Fig. 4a–e and Supplementary Fig. S3 ), which, on the basis of distinct morphological features, including: spherical/ovoidal cells adhering to >100 μm-long stalk appendages, tubular forks ( Fig. 4a–c ), exospore-like features ( Fig. 4b ) and fossilization mechanism, we interpret as fossil relatives of the anoxygenic photoferrotroph, Rhodomicrobium vanielii [7] , [8] , [23] , [24] . Similar to their modern counterparts, these microorganisms grew by polar budding, forming vast networks of cells connected end-to-end by stalk appendages, when transforming Fe 2+ to Fe 3+ during anoxygenic photosynthesis. The fossil structures are encrusted with haematite, the only oxyhydro(oxide) present on these biological structures and as free deposits ( Fig. 4f ). The predominance of haematite points to circumneutral depositional/diagenetic conditions, where haematite tends to be abundant between pH 7 and 8, with ferrihydrite as the precursor [25] . 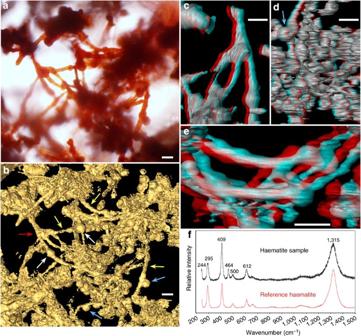Figure 4: Fossilized cells and stalks in specimen SMNH X5036. (a) Light micrographs of definitive photoferrotrophic features. (b) SRXTM isosurface rendering of panela. (c–e) SRXTM stereo anaglyphs (threshold-selected) surface renderings of parts of the same volume, showing: (c) tubular fork (red arrow). (d)R. vanieliiexospore-like structure (blue arrow). (e) Bunch of cells and stalks (white and yellow arrows, respectively). For detailed 3D visualization, use a pair of red–cyan or red–blue 3D glasses. Further details can be seen in Supplementary Movies 1 and 2. (f) Raman spectrum of encrusting iron-rich material identified as haematite, compared with a reference spectrum, RRUFF ID: R050300, from the RRUFF project39. The Raman band at 464 cm−1is from silica. Scale bar, 10 μm. Figure 4: Fossilized cells and stalks in specimen SMNH X5036. ( a ) Light micrographs of definitive photoferrotrophic features. ( b ) SRXTM isosurface rendering of panel a . ( c–e ) SRXTM stereo anaglyphs (threshold-selected) surface renderings of parts of the same volume, showing: ( c ) tubular fork (red arrow). ( d ) R. vanielii exospore-like structure (blue arrow). ( e ) Bunch of cells and stalks (white and yellow arrows, respectively). For detailed 3D visualization, use a pair of red–cyan or red–blue 3D glasses. Further details can be seen in Supplementary Movies 1 and 2. ( f ) Raman spectrum of encrusting iron-rich material identified as haematite, compared with a reference spectrum, RRUFF ID: R050300, from the RRUFF project [39] . The Raman band at 464 cm −1 is from silica. Scale bar, 10 μm. Full size image Most aerobic iron-oxidizing appendage bacteria escape entombment during growth on iron by discarding their stalks [26] , which probably explains why it is common to identify such structures in ancient sedimentary iron-rich rocks without associated cells [27] . However, R. vanielii becomes completely encrusted during anaerobic phototrophic growth on Fe, leading to the arrest of cell growth and Fe metabolism [7] , [8] . This probably accounts for the remarkable preservation we report here and for the fact that the cells and their stalks were heavily encrusted by haematite. Three major mechanisms are currently implicated in the oxidation of Fe 2+ to Fe 3+ : abiotic O 2 precipitation [1] , [26] , UV-driven photochemical Fe 2+ oxidation [1] , [2] and microbial transformation [1] , [3] , [6] , [7] , [8] , [9] , [10] , [11] , [12] , [13] , [14] , [28] . In addition to the low Archaean O 2 levels, recent experimental studies have rejected photochemical Fe 2+ oxidation as a potential major contributor to BIF formation [1] , [3] . Instead, it has been suggested through microbial culture studies and biogeochemical extrapolations that BIF deposition in the stratified Precambrian iron-rich oceans was entirely possible under the activity of the iron-oxidizing bacteria [1] , [3] , especially with the involvement of anoxygenic photoferrotrophs [12] , [13] , [14] . However, it has never been demonstrated in the natural environment how this was possible—that is, microbial transformation of Fe 2+ →Fe 3+ →BIFs—or how the activity of these microorganisms could have accounted for the alternating bands. In fact this process has never been shown to form BIFs, not in nature or in the laboratory. We show that the fossilized haematite-encrusted structures formed three-dimensional skeletons that tethered the iron-rich sections of the rock ( Fig. 4 and Supplementary Fig. S3 ), which can be better visualized with 3D visual aids in the synchrotron radiation X-ray microscopy tomographic stereo renderings presented in Fig. 3c–e , and Supplementary Movies 1 and 2 give a deeper appreciation of depth. We did not observe such geometries in portions of the rock populated by single cells, suggesting that a strong prerequisite for the formation of these 3D micro-fabrics was that the cells were immobilized in the stalk production phase and fossilized in their original spatial position, which is possible with R. vanielii [7] , [8] . In a stratified ocean, these photoferrotrophic biofilm gels would have formed below the chemocline, its depth and size dependent on light penetration. Following biofilm encrustation and death, soluble Fe 2+ in this zone would have remained suspended in the anoxic water column in the absence of any major oxidant. Continuous hydrothermal venting would have increased this soluble Fe 2+ pool, until a new biofilm succession became available to precipitate this soluble Fe 2+ pool to Fe 3+ . Cyclic lapse in intense photoferrotrophic Fe 2+ oxidation would have enabled the precipitation of the silica-rich bands, relative to the ratio of silica to Fe 2+ oxidized ( Fig. 5a ). This model is consistent with the fact that dense fossil biofilm populations encrusted with haematite tended to alternate with the chert-rich bands, which mostly lacked dense biofilms characteristic of the photoferrotrophic fossils and with lower haematite content ( Fig. 5b ). These in situ observations implicate biofilm density in both banding visibility and biogeochemistry. Nonetheless, the persistent high concentration of silica even in the iron-rich bands suggests that the silica load in the water column was probably constant, but that the rate of Fe 3+ precipitation determined the ratios of silica to iron deposited in the various bands. Therefore silica precipitation and sedimentation rates were probably much slower than biological Fe 3+ formation. These results demonstrate that cyclic growth and death of biofilms, after encrustation, allowed the incorporation of different ratios of silica and iron in the alternating bands ( Figs 3a and 5 ). 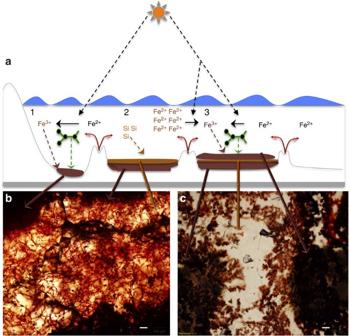Figure 5: A simplified model for photoferrotrophic deposition of banded iron rocks. (a) Intense phototrophic oxidation of hydrothermal Fe2+precipitates Fe3+together with microbial cells and stalks following biofilm (green lines connected by black filled rings) encrustation and death (1). Negative feedback halts Fe2+transformation to Fe3+allowing for the precipitation of Si, as most of the highly soluble Fe2+is retained in solution (2). Another episode of abundant photoferrotrophic biofilm growth and Fe3+encrustation leads to the deposition of a new iron-rich band (3). (b,c) Light micrographs showing direct environmental evidence for the proposed model. The two panels show examples of photoferrotrophic bacterial fossilization patterns related to the alternating Fe3+and silica precipitation in the Cape Vani rock deposits. Scale bar, 100 μm. Figure 5: A simplified model for photoferrotrophic deposition of banded iron rocks. ( a ) Intense phototrophic oxidation of hydrothermal Fe 2+ precipitates Fe 3+ together with microbial cells and stalks following biofilm (green lines connected by black filled rings) encrustation and death (1). Negative feedback halts Fe 2+ transformation to Fe 3+ allowing for the precipitation of Si, as most of the highly soluble Fe 2+ is retained in solution (2). Another episode of abundant photoferrotrophic biofilm growth and Fe 3+ encrustation leads to the deposition of a new iron-rich band (3). ( b , c ) Light micrographs showing direct environmental evidence for the proposed model. The two panels show examples of photoferrotrophic bacterial fossilization patterns related to the alternating Fe 3+ and silica precipitation in the Cape Vani rock deposits. Scale bar, 100 μm. Full size image Additionally, if photoferrotrophy was the main mechanism for Fe 3+ precipitation in the ancient oceans, variations in solar irradiation, including changes in Earth’s orbital eccentricity and obliquity, all of which influence water temperatures, light penetration and depth of the thermocline, would have caused strong temporal and spatial variations in intense photoferrotrophic Fe 3+ precipitation [28] . Experimental evidence suggests that low temperatures indeed promote Si precipitation over microbial Fe 2+ transformation and vice versa [29] . We suggest that cyclic blooming of anoxygenic photoferrotrophy, related to Fe 2+ oxidation followed by rapid encrustation and fossilization by Fe 3+ , is key to BIF formation and banding ( Fig. 5 ). It is possible that with the emergence of oxygen oases in the Archaean oceans [30] , [31] , [32] , [33] , [34] , [35] and the rise of atmospheric oxygen during the Great Oxidation Event (GOE), ~2.45 billion years ago [5] , rapid abiotic transformation of Fe 2+ to Fe 3+ by oxygen could have contributed to significant BIF formation [31] . This is feasible, especially if iron had a continental source, or if Fe 2+ upwelling from submarine hydrothermal sources reached the oxic surface waters above the chemocline. However, it has been suggested that in the redox-stratified Proterozoic oceans, following the GOE, anoxygenic photoferrotrophic activity below the chemocline might have hindered or reduced the potential contact of submarine-derived Fe 2+ with the overlying oxic surface waters [14] . Specifically, an origin below the chemocline of late Palaeoproterozoic BIFs has been suggested—implicating biotic processes in their formation [4] . Our model supports and is favoured by these various hypotheses. Furthermore, the Archaean BIFs were deposited under anaerobic conditions, where anoxygenic photoferrotrophy activity was probably important [4] , [36] . The high demand for oxygen required for the abiotic deposition of BIFs at the scale recorded in the anoxic Archaean world is problematic. Proponents of biological processes linked to the oxygen deposition model suggest that primitive Archaean oxygenic photosynthetic bacteria thrived during periodic Fe 2+ availability [36] , [37] , supplying oxygen to microaerophilic Fe 2+ oxidizers capable of precipitating Fe 3+ (ref. 38 ). Although feasible, clear in situ evidence for this process or the scale of it and what caused the proposed periodicity in iron availability is lacking. Band development in BIFs has been related to basinal silicification due to evaporitic and climatic fluctuations [1] , whereas periodic volcanism is said to have increased oceanic hydrothermal iron flux [1] , [4] , [38] . The latter process supports our hypothesis for a hydrothermal origin of the Cape Vani BIF analogues. However, combined, these suggestions do not reliably account for the periodicity of the fine, alternating BIF banding texture. Neither do they explain why iron would be preferentially sedimented over silica and vice versa . As we have demonstrated, microorganisms, when coupled to our model, could easily have controlled both the deposition of BIFs and band formation at different scales. Conveniently, the scale of their activity could have been coupled to increased volcanic release of iron and climatic fluctuations. Microbial growth cycles are universally affected by changes in environmental conditions—including nutrient availability and temperatures [28] , [29] . A scenario much difficult to explain involves the role of microaerophilic iron oxidizers in vast deposition of Archaean BIFs. These microorganisms have a high requirement for oxidizing huge quantities of iron to generate small amounts of cellular energy [26] . As a consequence, a persistent and tremendous oxygen supply source would have been required over the course of this entire process to enable large-scale BIF formation in the predominantly anoxic Archaean oceans. Perhaps oxygen exerted a stronger impact on BIF formation after the GOE, through both abiotic rapid oxygen precipitation of iron and biotic microaerophilic bacterial iron oxidation [4] , [19] . At this time, the oceans had become stratified and predominated by deep-water reducing conditions. Our model provides a clear example of how anaerobic biological processes might have continued to contribute towards BIF deposition below the chemocline, in the presence of an elevated oxygen atmosphere and overlying oxic surface waters. This would have been the case, especially if the oceans were relatively calm. As we show, the Cape Vani BIF analogue was deposited under anoxic conditions, below an atmosphere of present-day atmospheric oxygen concentrations. It is thus likely that with lesser oxygen levels present in the early Archaean/Palaeoproterozoic oceans, this process might have been able to contribute to significant BIF deposition. There is evidence of a chemocline reaching >100 m depth already by 2.5 Ga [19] , [33] and the ability of anoxygenic photoferrotrophs to utilize light in the wavelengths reaching this depth [14] . It is therefore possible that these microorganisms could have formed vast and uninterrupted biofilms just below this layer, enough to generate extensive BIF deposits. In addition, biological Fe 3+ precipitation involves both active and passive processes [26] . Thus, in the case where surplus Fe 3+ was being precipitated by oxygen in the overlying oxic surface waters, it could have been passively adsorbed by the biofilms below the chemocline during Fe 3+ rain-down. Such an alternate hypothesis could still be explained by our banding model, if the encrusted and denser biofilms sedimented faster. This model is possible, particularly if iron supply to the oxic surface waters occurred in pulses. However, our data show no evidence for this process. The Cape Vani BIF depositional conditions are similar to those in the early oceans, but the basin was limited in size—laterally (~1 km) and probably vertically too (depth, unknown)—compared with superior-type BIF deposits, stretching hundreds of kilometres. In the predominantly oxic Early Quaternary atmosphere, the small scale of this basin would have exerted a major force on the development of typical Precambrian ocean conditions (suitable redox and adequate levels of silica and iron concentrations) over extended periods. In the largeness of the open ocean, these circumstances, which probably influenced band periodicity and thickness, would have been diluted. Hence we assume this basin to be a scaled-down version of the Precambrian oceans, where processes were also scaled down accordingly. The Cape Vani deposits and their microbial fossils are extremely well preserved, with apparently no regional contact deformation and metamorphism [15] , [16] , making them a remarkable new analogue system for unravelling the in situ biogeochemical processes that might have orchestrated the large-scale deposition of BIFs. If indeed these are young BIF analogues, then the geochemical data provide new insights on the probable chemical constitution of BIFs prior to diagenesis, deformation and metamorphism, billions of year later. We conclude that anoxygenic photoferrotrophy might have had a crucial role in the biogeochemical transformation of the early geobiosphere and that microbial activity and their fossilization mechanisms are not only directly implicated in iron-oxyhydro(oxides) deposition, but might have also been vital for the formation of micro-fabrics that enhanced the structural integrity of BIFs. Optical microscopy Reflected light microscopy and imaging was performed on doubly polished sections (~150–200- μm-thick) with an Olympus BX51 microscope fitted with an Olympus DP71 camera. Images were acquired using the Olympus cellSens 1.7 Digital Imaging software. Raman spectroscopy The thin sections were analysed with a laser Raman confocal spectrometer (Horiba instrument LabRAM HR 800), equipped with a multichannel air-cooled charge-coupled device detector and an Ar-ion laser ( l =514 nm) as the excitation source. A power output of 8 mW was focused on the sample. The instrument was integrated with an Olympus BX51 microscope. The wavelength of the laser beam focused on 1μm specimen spots with a × 100 objective was changed from l =514 nm to λ =514 nm and the diameter from 1 mm to μm. The spectral resolution was ~0.3 cm −1 . The instrument was calibrated with a neon lamp and the Raman line (520.7 cm −1 ) of a silicon wafer. Instrument control and data acquisition were made using LabSpec 5 software. Synchrotron radiation X-ray tomographic microscopy Thin sections were reduced in size and mounted on a 3-mm-wide brass peg and analysed on the TOMCAT beamline at the Swiss Light Source at the Paul Scherrer Institute [39] , [40] . The X-ray energy was optimized for maximum contrast at 13–20 keV. A total of 1501 projections were acquired equiangularly over 180°, post-processed online and rearranged into flat- and darkfield-corrected sinograms. Reconstruction was performed on a Linux PC farm using highly optimized routines based on the Fourier Transform method [40] . A × 20 lens was used, resulting in stacks with a voxel size of 0.37 μm. The data derived from the scans were then analysed and rendered using Avizo ( http://www.vsg3d.com/ ) software. Elemental analysis of rock samples AcmeLabs ( http://acmelab.com ) conducted analyses on 0.2 g of whole rock samples. Eu/Eu* and Ce/Ce* anomalies were calculated using the NASC reference standard as previously described for BIFs [41] . Sample storage The microbial fossil specimens are deposited at the Swedish Museum of Natural History under the reference numbers: SMNH X5036 and SMNH X5037. The sawn rock samples are deposited at the Museum of Palaeontology and Geology, National and Kapodistrian University of Athens and given reference numbers: AMPG 936 and AMPG 935. How to cite this article: Chi Fru, E. et al. Fossilized iron bacteria reveal a pathway to the biological origin of banded iron formation. Nat. Commun. 4:2050 doi: 10.1038/ncomms3050 (2013).